Holey graphene frameworks for highly efficient capacitive energy storage Supercapacitors represent an important strategy for electrochemical energy storage, but are usually limited by relatively low energy density. Here we report a three-dimensional holey graphene framework with a hierarchical porous structure as a high-performance binder-free supercapacitor electrode. With large ion-accessible surface area, efficient electron and ion transport pathways as well as a high packing density, the holey graphene framework electrode can deliver a gravimetric capacitance of 298 F g −1 and a volumetric capacitance of 212 F cm −3 in organic electrolyte. Furthermore, we show that a fully packaged device stack can deliver gravimetric and volumetric energy densities of 35 Wh kg −1 and 49 Wh l −1 , respectively, approaching those of lead acid batteries. The achievement of such high energy density bridges the gap between traditional supercapacitors and batteries, and can open up exciting opportunities for mobile power supply in diverse applications. Electrochemical capacitors (ECs), also known as supercapacitors, represent an attractive technology for energy storage and mobile power supply. ECs typically exhibit superior power density and cycle life, but with relatively poor energy density at least one order of magnitude lower than those of traditional batteries [1] , [2] , [3] . The electrode material is the central component of an EC and largely dictates its ultimate performance. Considerable efforts have been focused on developing new electrode materials that can greatly increase the energy density without sacrificing the power density or cycle life [3] , [4] , [5] , [6] . In general, a high-performance EC electrode requires high electrical conductivity, high ion-accessible surface area, high ionic transport rate and high electrochemical stability. To this end, carbon-based porous materials represent the most attractive class of EC electrode materials. The state-of-the-art ECs available today are mainly constructed using porous activated carbon electrodes typically with a gravimetric capacitance of 80–120 F g − 1 and a stack energy density of 4–5 Wh kg − 1 (ref. 4 ), much lower than that of lead acid batteries (25–35 Wh kg −1 ) (ref. 1 ). Graphene has recently received intensive interest as a new EC electrode material because of its high intrinsic electrical conductivity, excellent mechanical flexibility, exceptionally large theoretical surface area of 2,630 m 2 g −1 and theoretical gravimetric capacitance of about 550 F g −1 (refs 7 , 8 ). However, due to the strong π – π interaction between graphene sheets, the graphene flakes tend to restack to form graphite-like powders or films, which can severely decrease the accessible surface area and reduce the ion diffusion rate, resulting in unsatisfactory gravimetric capacitances (typically <180 F g −1 in organic electrolytes) and relatively low charge/discharge rates [7] , [8] , [9] , [10] , [11] . A traditional activation method was recently employed to prepare activated graphene with abundant ultrasmall micropores and ultrahigh specific surface area up to 2,400–3,100 m 2 g −1 (ref. 12 ), but only with a gravimetric capacitance of 165 F g −1 because of the difficulty for the electrolyte ions to efficiently access the micropore surfaces [3] . More recently, it has been shown that laser-scribed graphene with open porous structure can be used to mitigate these challenges to increase the accessible surface area and boost the gravimetric capacitance up to 276 F g −1 (ref. 13 ). Although gravimetric capacitance was traditionally used as the figure-of-merit to evaluate an EC electrode, the volumetric performance is becoming an increasingly important metric to consider for many practical applications with limited space such as portable electronic products [14] , [15] , [16] , [17] , [18] , [19] , [20] . However, there is usually a trade-off relationship between the gravimetric and volumetric capacitances for most electrode design. On one hand, a highly porous electrode can offer large specific surface area and favour ion diffusion for high gravimetric capacitance, but usually results in a lower volumetric capacitance due to its relatively low packing density. In addition, an EC electrode made from low-packing-density materials usually have abundant empty spaces that could be flooded by the electrolyte, which could increase the total mass of the device and lower the overall energy density normalized by the total mass of the entire device [14] , [15] . On the other hand, a more compact electrode may boost the volumetric capacitance but decrease the ion-accessible surface area and ion diffusion rate to result in a lower gravimetric capacitance and poor rate performance. For example, for the EC electrodes made from laser-scribed porous graphene aforementioned, they typically exhibit a rather low packing density of ~0.05 g cm −3 , and consequently a relatively low volumetric capacitance in spite of their excellent gravimetric performance [13] . By creating a highly compact graphene film using vacuum filtration and capillary compression, a recent study has reported a greatly improved volumetric capacitance exceeding 200 F cm −3 , yet with a modest gravimetric capacitance of 167 F g −1 (ref. 16 ). Together, it remains a considerable challenge to simultaneously achieve high gravimetric and high volumetric capacitances while retaining excellent rate capability. Here, we report a free-standing holey graphene framework (HGF) with a high packing density and efficient ion transport pathway to enable high-performance EC electrodes simultaneously with the highest gravimetric capacitance (298 F g −1 ) and the highest volumetric capacitance (212 F cm −3 ) achieved in organic electrolyte to date. We further show that a fully packaged HGF EC can deliver gravimetric and volumetric energy densities of 35 Wh kg −1 and 49 Wh l −1 , approaching those of lead acid batteries. Structural features of HGFs for supercapacitors The HGFs are formed by conjugating holey graphene sheets into a free-standing three-dimensional (3D) network. The unique structure of the HGFs satisfies several critical requirements for an ideal EC electrode ( Fig. 1 ). First, the graphene sheets in 3D network are highly interconnected and interlocked together to prevent them from restacking and to maintain a highly porous monolithic graphene framework (GF) ( Fig. 1a ) with large specific surface area (around 1,030 m 2 g −1 based on methylene blue (MB) adsorption), and the creation of nanopores in holey graphene sheets ( Fig. 1b ) can further boost the specific surface area up to 1,560 m 2 g −1 . Second, the HGFs are initially fully hydrated and can allow direct exchange of various electrolytes to ensure the entire surface area fully wetted by the electrolyte and accessible by electrolyte ions and thus electrochemically active, which is difficult to achieve in conventional porous carbon material [3] , [15] or recently reported activated graphene [12] . Third, the solvated HGFs with interlocked graphene sheets can be mechanically compressed to form free-standing compact HGF films ( Fig. 1c,d ) without complete restacking to achieve a high packing density of 0.71 g cm −3 while maintaining the initial solvated condition. The HGF films exhibit excellent electrical conductivity (~1,000 S m −1 ) about one to two orders of magnitude higher than that of activated carbon (10–100 S m −1 ) (ref. 21 ) and also two times better than that of activated graphene (500 S m −1 ) (ref. 12 ), and thus can be used as EC electrodes directly. Lastly, unlike the ultrasmall micropores in activated graphene that are difficult to be accessed by electrolyte ions, the pores in HGFs are sufficiently large and well integrated into a hierarchical porous architecture to form a highly continuous network of open channels for efficient ion transport throughout the entire network even under the highly compressed form. In particular, the nanopores in holey graphene sheets are large enough to function as the ion diffusion shortcuts between different layers of graphene to greatly speed up the ion transport across the entire film and facilitate ion access to the entire surface area ( Fig. 1f ), which is not possible with non-holey GFs ( Fig. 1e ). Together, these combined features make it possible for HGFs to achieve high volumetric capacitance while retaining high gravimetric capacitance and excellent rate capability. 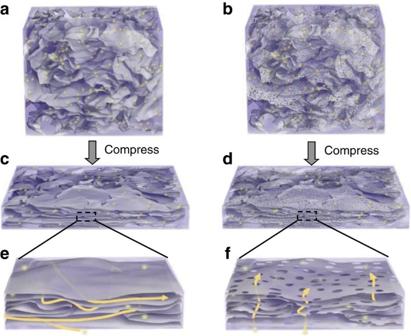Figure 1: Schematic illustration of the HGFs as an ideal material for EC electrodes. (a,b) Initial solvated 3D macroporous structures of GFs (a) and HGFs (b). (c,d) Compressed films of the solvated GFs (c) and HGFs (d). (e,f) A closed-up view of GF (e) and HGF (f) films, with the arrows highlighting the ion transport pathway. The ions in GF film need to travel much longer distance to find the broken edge of graphene sheet to cross each layer of graphene sheet in the GF film, while the nanopores in holey graphene sheet of HGF can function as the ion transport shortcuts between neighbouring layers of graphene to greatly speed up the ion transport across the entire HGF film. Figure 1: Schematic illustration of the HGFs as an ideal material for EC electrodes. ( a , b ) Initial solvated 3D macroporous structures of GFs ( a ) and HGFs ( b ). ( c , d ) Compressed films of the solvated GFs ( c ) and HGFs ( d ). ( e , f ) A closed-up view of GF ( e ) and HGF ( f ) films, with the arrows highlighting the ion transport pathway. The ions in GF film need to travel much longer distance to find the broken edge of graphene sheet to cross each layer of graphene sheet in the GF film, while the nanopores in holey graphene sheet of HGF can function as the ion transport shortcuts between neighbouring layers of graphene to greatly speed up the ion transport across the entire HGF film. Full size image Preparation and characterization of HGFs The HGFs were prepared through a one-step process with simultaneous low-temperature etching of nanopores in graphene and self-assembly of graphene into 3D network structures ( Fig. 2a ). A controlled amount of H 2 O 2 aqueous solution was added into a well-dispersed graphene oxide (GO) aqueous dispersion. The mixture was sealed in a Teflon-lined autoclave and heated at 180 °C for 6 h to yield mechanically strong monolithic HGFs ( Fig. 2b ). During the hydrothermal process, GO sheets were reduced ( Supplementary Fig. 1 ) and self-assembled into hydrogels with interconnected 3D macroporous network ( Fig. 2c ) with the pore sizes ranging from sub-micrometres to several micrometres and the pore walls consisting of single- or few-layer graphene sheets ( Supplementary Fig. 2 ) [22] , [23] , [24] , [25] . At the same time, H 2 O 2 molecules can partially oxidize and etch the carbon atoms around the more active defective sites of GO, leaving behind carbon vacancies, which gradually extend into nanopores [26] . Since the defective carbon sites are generally distributed throughout the basal plane of GO [27] , the etching process could occur across the entire graphene sheets to result in abundant in-plane pores of a few nanometres ( Fig. 2d and Supplementary Fig. 3 ). In control experiments without adding H 2 O 2 , GFs consisting of non-holey graphene sheets ( Fig. 2e ) are obtained, consistent with previous studies [22] . Furthermore, excessive H 2 O 2 would lead to a more aggressive etching, enlarging the pore size of holey graphene and breaking them into small pieces ( Supplementary Fig. 4 ). As a result, the HGFs become very fragile and unsuitable for binder-free EC electrodes. Nitrogen adsorption-desorption tests showed the freeze-dried HGF had a Brunauer–Emmett–Teller (BET)-specific surface area of 830 m 2 g −1 , which is significantly larger than that of non-holey GF (~260 m 2 g −1 ) ( Supplementary Fig. 5a,b ). Because the freeze drying used to prepare BET sample can induce partial restacking of some graphene layers and reduce the apparent specific surface area, we have also used MB adsorption method to more accurately determine the solvated surface area of the HGF to be 1,560 m 2 g −1 and that of non-holey GF to be 1,030 m 2 g −1 . 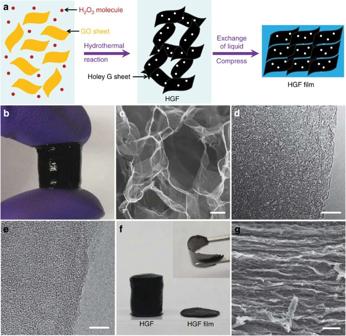Figure 2: Preparation and structural characterization of HGFs. (a) Schematic illustration of the preparation process of HGFs and HGF films. (b) A photograph showing a free-standing HGF. (c) Scanning electron microscope image of interior microstructures of HGFs. Scale bar, 1 μm. (d) Transmission electron microscopy (TEM) image of holey graphene sheets in HGFs. Scale bar, 10 nm. (e) TEM image of non-holey graphene sheets in GFs for comparison. Scale bar, 10 nm. (f) A photograph showing HGFs before and after mechanical compression with the flexibility of the compressed HGF film shown in the inset. (g) Cross-sectional SEM image of the compressed HGF film. Scale bar, 1 μm. Figure 2: Preparation and structural characterization of HGFs. ( a ) Schematic illustration of the preparation process of HGFs and HGF films. ( b ) A photograph showing a free-standing HGF. ( c ) Scanning electron microscope image of interior microstructures of HGFs. Scale bar, 1 μm. ( d ) Transmission electron microscopy (TEM) image of holey graphene sheets in HGFs. Scale bar, 10 nm. ( e ) TEM image of non-holey graphene sheets in GFs for comparison. Scale bar, 10 nm. ( f ) A photograph showing HGFs before and after mechanical compression with the flexibility of the compressed HGF film shown in the inset. ( g ) Cross-sectional SEM image of the compressed HGF film. Scale bar, 1 μm. Full size image With the highly porous structure and excellent mechanical stability, the as-prepared HGF can be greatly compressed using a hydraulic press to form a free-standing compact HGF film with nearly 60-fold increase in packing density. For example, a piece of ~1-cm thick HGF with a packing density of ~12 mg cm −3 can be compressed to a ~140-μm thick flexible film with a packing density of ~0.71 g cm −3 ( Fig. 2f,g ). X-ray diffraction studies of HGFs before and after compression showed similar diffraction peak width and intensity, suggesting the initial arrangement between graphene sheets in HGFs was not obviously altered by compression ( Supplementary Fig. 2 ). Meanwhile, the compressed HGF films exhibited a BET specific surface area of ~810 m 2 g −1 , close to that of uncompressed HGFs (~830 m 2 g −1 ; Supplementary Fig. 5c,d ), further suggesting that little restacking is occurring in the compressed HGF films. This can be attributed to the robust interlock of graphene sheets that allows mechanical compression to reduce the pore size without significantly modifying the stacking characteristics of graphene and its 3D interconnected porous structure [18] . Importantly, these compressed HGF films can exhibit excellent electrical conductivity of ~1,000 S m −1 , and are mechanically strong enough to be used as the EC electrodes directly. To explore the potential of HGFs for capacitive energy storage, we have fabricated a series of symmetric HGF-based ECs (HGF-ECs) using the compressed HGF films as both electrodes and investigated their electrochemical characteristics in aqueous and organic electrolytes. The areal mass loading of HGF in one electrode is about 1 mg cm −2 of graphene. As a control experiment, compressed non-holey GF films were also used to create GF-ECs. All electrochemical results below are based on the compressed HGF and GF films unless otherwise specified. Electrochemical performance of HGFs in aqueous electrolyte The cyclic voltammetry (CV; Fig. 3a ) and galvanostatic charge/discharge studies ( Fig. 3b ) showed a greatly enhanced electrochemical performance for HGF-ECs in comparison with GF-ECs. The nearly rectangular CV curves at a high scan rate of 1,000 mV s −1 and the nearly triangular charge/discharge curves at a high current density of 100 A g −1 indicate a nearly ideal electrical-double-layer capacitive behaviour and efficient electrolyte ion transport throughout the HGF electrodes. A weak pair of broad peak seen in CV curve is probably due to a minor contribution from the redox reaction of residual oxygen-containing groups on the graphene sheets of HGF [25] . In addition, it is evident that HGF-EC exhibited a smaller voltage drop ( IR drop) of 0.12 V than GF-EC (0.26 V) at the start point of the discharge curves ( Fig. 3b ), from which we can derive the equivalent series resistance (ESR) of 0.6 and 1.3 Ω for the HGF-EC and GF-EC, respectively. The specific capacitance values can be derived from charge/discharge curves ( Fig. 3c ). The HGF electrodes exhibited an ultrahigh gravimetric capacitance of 310 F g −1 at a current density of 1 A g −1 . In contrast, the gravimetric capacitance of non-holey GF electrodes is about 208 F g −1 at 1 A g −1 . On increasing the current density up to 100 A/g, the HGF electrodes retained about 76% of its initial capacitance (237 F g −1 ), while the non-holey GF only showed a 63% capacitance retention (131 F g −1 ). 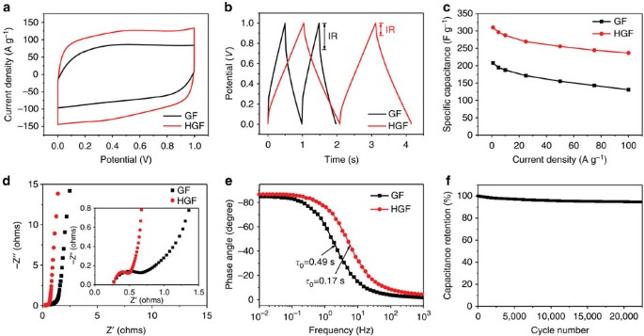Figure 3: Electrochemical characterization of HGF-EC and GF-EC in 6 M KOH. (a) CV curves of HGF-EC and GF-EC at a high scan rate of 1,000 mV s−1. (b) Galvanostatic charge/discharge curves of HGF-EC and GF-EC at a high current density of 100 A g−1. (c) Comparison of specific capacitances versus different current densities for HGF-EC and GF-EC. (d) Nyquist plots of HGF-EC and GF-EC. The inset shows the close-up view of the high-frequency regime. (e) Bode plots of phase angle versus frequency. (f) Cycling stability of HGF-EC at a current density of 25 A g−1. Figure 3: Electrochemical characterization of HGF-EC and GF-EC in 6 M KOH. ( a ) CV curves of HGF-EC and GF-EC at a high scan rate of 1,000 mV s −1 . ( b ) Galvanostatic charge/discharge curves of HGF-EC and GF-EC at a high current density of 100 A g −1 . ( c ) Comparison of specific capacitances versus different current densities for HGF-EC and GF-EC. ( d ) Nyquist plots of HGF-EC and GF-EC. The inset shows the close-up view of the high-frequency regime. ( e ) Bode plots of phase angle versus frequency. ( f ) Cycling stability of HGF-EC at a current density of 25 A g −1 . Full size image We have further probed the ion transport properties within the HGFs using electrochemical impedance spectroscopy (EIS). A frequency response analysis over the frequency range from 100 kHz and 10 mHz yields the Nyquist plots ( Fig. 3d ). The plot features a vertical curve in low-frequency regime, indicating a nearly ideal capacitive behaviour. A close-up observation of the high-frequency regime reveals a transition from a vertical curve to a 45° Warburg region followed by a semicircle ( Fig. 3d , inset). The HGF-EC exhibits a shorter 45° region and smaller diameter semicircle, indicating a lower charge transfer resistance and more efficient electrolyte diffusion within the HGF electrodes [6] . By extrapolating the vertical portion of the plot to the real axis, an ESR of 0.65 and 1.25 Ω was obtained for HGF-EC and GF-EC, respectively, consistent with the galvanostatic charge/discharge studies ( Fig. 3b ). It should be noted that the ESR of an EC is related to both electrical resistance of the electrodes and ion diffusion resistance in the electrodes [5] . Although the GF film has a better conductivity than HGF film (~1,400 S m −1 versus ~1,000 S m −1 ), the HGF film has a much better ion diffusion property ( Fig. 3d ), leading to a lower ESR and a smaller IR drop in the charge/discharge curves of HGF-EC. The dependence of phase angle on the frequency for the HGF-EC and GF-EC shows that the phase angles of both devices are close to −90° at low frequencies, confirming an ideal capacitive behaviour ( Fig. 3e ). The characteristic frequency f 0 at a phase angle of −45° marks the point where the resistive and capacitive impedances are equal [28] . The HGF-EC and GF-EC exhibit an f 0 of 5.88 Hz and 2.04 Hz, respectively, which corresponds to a time constant τ 0 (=1/ f 0 ) of 0.17 s for HGF-EC, about one-third of that of GF-EC (0.49 s) and greatly lower than those of conventional activated carbon-based ECs (10 s) (ref. 13 ). This rapid frequency response of HGF-EC further suggests the significantly enhanced ion transport rate within the HGF electrodes. The cycling test of HGF-EC showed 95% capacitance retention over 20,000 cycles at a high current density of 25 A g −1 ( Fig. 3f ), demonstrating excellent electrochemical stability of the device. These studies demonstrate that the HGF electrodes not only exhibit much higher specific capacitances than GF electrodes, but also show greatly improved rate capability and capacitance retention at high charging/discharging rate, which can be attributed to higher ion-accessible surface area and more rapid ion transport in the unique hierarchical porous network of HGFs (see Fig. 1e,f ). Electrochemical performance of HGFs in organic electrolyte Since energy stored in an EC is proportional to the square of voltage, organic electrolytes are usually more desirable for ECs due to their wider electrochemical window as compared with aqueous electrolytes. To this end, we have further tested the electrochemical performance of HGF-ECs in 1-ethyl-3-methylimidazolium tetrafluoroborate/acetonitrile (EMIMBF 4 /AN) electrolyte. The CV testing showed rectangular curves from 0 to 3.5 V even at a high scan rate of 500 mV s −1 ( Fig. 4a ). Meanwhile, galvanostatic charge/discharge curves showed a nearly symmetric triangular shape with small voltage drops at the initial point of the discharge curve (0.26 V at the current density of 50 A g −1 ; Fig. 4b ). Both results suggest an excellent electrical-double-layer capacitive behaviour and a very low ESR (2.6 Ω) in HGF-EC. Three-electrode CV test at a low scan rate of 5 mV s −1 ( Supplementary Fig. 6 ) showed there was little pseudocapacitance contribution. The HGF electrodes showed an impressive gravimetric capacitance of 298 F g −1 at a current density of 1 A g −1 ( Fig. 4c ), only about 4% lower than that in aqueous electrolyte (310 F g −1 ). Increasing the current density to 100 A g −1 , the HGF electrodes retained a high gravimetric capacitance of 202 F g −1 . The achievement of such high gravimetric capacitances in organic electrolyte (298 F g −1 ) leads to an unprecedented gravimetric energy density of 127 Wh kg −1 ( Supplementary Table 1 ), which is nearly comparable to the theoretical value (165 Wh kg −1 ) of lead-acid battery electrodes [29] . On the basis of their packing density of 0.71 g cm −3 , the volumetric capacitance and energy density of HGF electrodes were calculated to be 212 F cm −3 and 90 Wh l −1 , respectively, also the best values achieved in all carbon-based EC electrodes to date ( Supplementary Table 1 ). 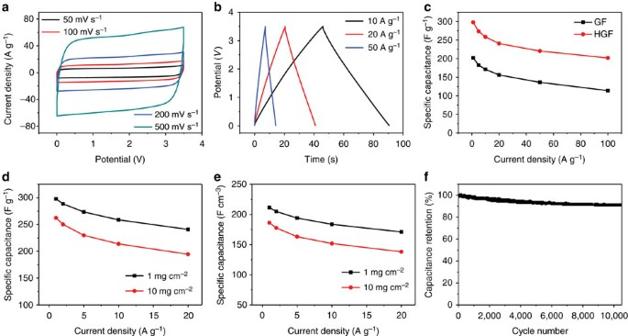Figure 4:Electrochemical characterization of HGF-EC in EMIMBF4/AN. (a,b) CV curves (a) and galvanostatic charge/discharge curves (b) of HGF-EC. (c) Comparison of specific capacitances of HGF and GF electrodes versus different current densities. (d,e) Gravimetric (d) and volumetric (e) capacitances of HGF electrodes versus different current densities (with graphene areal mass loading of 1 and 10 mg cm−2, respectively). (f) Cycling stability of HGF-EC at a current density of 20 A g−1. Figure 4: Electrochemical characterization of HGF-EC in EMIMBF 4 /AN. ( a , b ) CV curves ( a ) and galvanostatic charge/discharge curves ( b ) of HGF-EC. ( c ) Comparison of specific capacitances of HGF and GF electrodes versus different current densities. ( d , e ) Gravimetric ( d ) and volumetric ( e ) capacitances of HGF electrodes versus different current densities (with graphene areal mass loading of 1 and 10 mg cm −2 , respectively). ( f ) Cycling stability of HGF-EC at a current density of 20 A g −1 . Full size image To evaluate the practical potential of an EC device, it is particularly important to compare the energy density values (stack energy density) normalized by the total mass or volume of the entire EC stack that includes both electrodes, current collectors, electrolyte, separator (and packaging) instead of the active electrode materials alone [14] , [15] . To this end, it is necessary to increase the content of electrode materials (for example, areal mass loading of electrode materials) to increase active material ratio and maximize the stack energy density. However, this is not always straightforward since a thicker electrode can often increase ESR and decrease ion diffusion rate, leading to a rapid degradation in capacitive performances [30] , which can consequently limit the achievable stack energy density in a practical device. To evaluate the performance of our HGF electrodes for practical ECs, we have tested the electrochemical properties of much thicker HGF electrodes (140 μm in thickness) with an areal mass loading of ~10 mg cm −2 of graphene ( Supplementary Fig. 7 ), which is comparable to the carbon amount contained in many commercial ECs. Because of the high electrical conductivity and excellent ion diffusion within the HGF electrodes, the gravimetric capacitance of HGF electrode decreased by only 12% from 298 to 262 F g −1 at 1 A g −1 as the mass loading is increased from 1 to 10 mg cm −2 ( Fig. 4d ), with a slightly increased ESR of 3.6 Ω, which in turn yields a gravimetric energy density of 112 Wh kg −1 . Accordingly, the volumetric capacitance and volumetric energy density of HGF electrodes were slightly reduced to 186 F cm −3 ( Fig. 4e ) and 79 Wh L −1 , respectively. Both gravimetric and volumetric values are higher than previous reports for carbon-based materials including activated carbon [4] , carbon nanotubes [31] and graphene [10] , [11] , [12] , [16] with large areal mass loadings ( Supplementary Table 1 ). The HGF-EC with EMIMBF 4 /AN electrolyte also exhibited excellent cycling stability, with 91% of its initial capacitance retained after 10,000 charge/discharge cycles at a high current density of 20 A g −1 ( Fig. 4f ). This excellent cycling stability along with the three-electrode test ( Supplementary Fig. 6 ) suggest that the residual oxygen functionality plays a relatively minor role in the charge/discharge process and would not induce significant side reactions in organic electrolyte. It should be noted that although AN solvent is widely used for promoting the ion transport and rate performance [4] , [15] , the AN-based electrolyte is not suitable for the operation of ECs in high-temperature technical areas. Therefore, we have also conducted additional experiments to evaluate the energy density of our HGF electrode in neat EMIMBF 4 , which show nearly the same specific capacitance (289 F g −1 and 205 F cm −3 ) and energy densities (123 Wh kg −1 and 87 Wh l −1 ) ( Supplementary Fig. 8 ). The ability to achieve similar high capacitance without AN further demonstrates the unique advantage of HGF for efficient electrolyte transport and efficient surface area access, in contrast to previous studies. Comparison with the state-of-the-art devices To further evaluate the practical potential of our devices, we experimentally determined the stack energy density values which were normalized by the total mass or volume of the device including both electrodes, current collectors, electrolyte, separator (and packaging) ( Fig. 5a,b ). If excluding the packaging, the HGF electrodes account for ~37% weight of the device and thus our device delivers a high gravimetric and volumetric stack energy densities of 41.6 Wh kg −1 and 63.2 Wh l −1 , respectively ( Fig. 5b ). To include packaging, we used parafilm to seal our devices similarly to recent studies ( Fig. 5a ) [16] , and obtained a practical stack energy densities of 35.1 Wh kg −1 and 49.2 Wh l −1 for the fully packaged device, which are nearly one order of magnitude higher than those of commercial activated carbon-based ECs (4–5 Wh kg −1 and 5–7 Wh l −1 ) (ref. 4 ) and comparable to those of lead-acid batteries (25–35 Wh kg −1 and 50–90 Wh l −1 ) (ref. 1 ; Fig. 5c,d ). 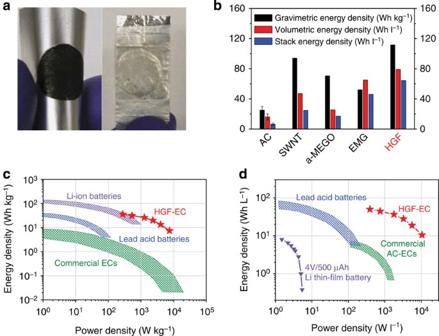Figure 5: Comparison of the energy and power densities of HGF-ECs with other state-of-art energy storage technologies. (a) Photographs of one HGF film electrode and one assembled symmetric HGF-EC. (b) Gravimetric and volumetric energy densities (normalized by the total weight or volume of both electrodes in each EC) and volumetric stack energy densities (normalized by the volume of the whole EC including two electrodes, two current collectors, electrolyte and one separator without packaging) for ECs made from various carbon materials. Areal mass loading of electrode materials: activated carbon (AC: 5 to 10 mg cm−2) (ref.4), single-walled carbon nanotube (5 mg cm−2) (ref.31), activated microwave exfoliated GO (2.5 mg cm−2) (ref.12), electrolyte-mediated graphene (10 mg cm−2) (ref.16), HGF (10 mg cm−2). (c) Ragone plots of gravimetric energy density versus gravimetric power density for HGF-EC in comparison with lead-acid batteries3, lithium-ion battery3, commercial ECs3. (d) Ragone plots of volumetric energy density versus volumetric power density for HGF-EC in comparison with lead-acid batteries1,3, lithium thin-film battery32, commercial activated carbon-ECs4,15. The energy and power densities are normalized by the actual weight or volume of the entire device stack including two electrodes, two current collectors, electrolyte, one separator and packaging. Figure 5: Comparison of the energy and power densities of HGF-ECs with other state-of-art energy storage technologies. ( a ) Photographs of one HGF film electrode and one assembled symmetric HGF-EC. ( b ) Gravimetric and volumetric energy densities (normalized by the total weight or volume of both electrodes in each EC) and volumetric stack energy densities (normalized by the volume of the whole EC including two electrodes, two current collectors, electrolyte and one separator without packaging) for ECs made from various carbon materials. Areal mass loading of electrode materials: activated carbon (AC: 5 to 10 mg cm −2 ) (ref. 4 ), single-walled carbon nanotube (5 mg cm −2 ) (ref. 31 ), activated microwave exfoliated GO (2.5 mg cm −2 ) (ref. 12 ), electrolyte-mediated graphene (10 mg cm −2 ) (ref. 16 ), HGF (10 mg cm −2 ). ( c ) Ragone plots of gravimetric energy density versus gravimetric power density for HGF-EC in comparison with lead-acid batteries [3] , lithium-ion battery [3] , commercial ECs [3] . ( d ) Ragone plots of volumetric energy density versus volumetric power density for HGF-EC in comparison with lead-acid batteries [1] , [3] , lithium thin-film battery [32] , commercial activated carbon-ECs [4] , [15] . The energy and power densities are normalized by the actual weight or volume of the entire device stack including two electrodes, two current collectors, electrolyte, one separator and packaging. Full size image The increase in the energy density of ECs usually comes at the cost of power density and/or cyclability, which are the most important characteristics of ECs and without which they become mediocre batteries [14] . With fast electron transport and efficient ion transport throughout the entire HGF film electrode, the HGF-EC could also deliver high power densities that are about one order of magnitude higher than those of commercial activated carbon-based ECs, more than two orders of magnitude higher than those of lead acid batteries and three orders of magnitude higher than that of the lithium thin-film batteries [32] ( Fig. 5c,d ). Unlike many studies in the community, in which the stack energy densities are often derived by extrapolation of rather small devices, our stack energy density is determined completely by experiments on practical devices with the size and mass comparable to commercial devices. With a large areal mass loading of HGF electrodes up to 10 mg cm −2 , our device shows an areal energy density of 22.4 Wh m −2 at an areal power density of 176 W m −2 , which exceeds those of commercial devices (2–6 Wh m −2 ) and laboratory devices (<16 Wh m −2 ) ( Supplementary Table 1 ). A typical packaged device with 1 cm 2 area can deliver a total energy of 2.24 mWh and power of 17.6 mW, also surpassing most previous studies ( Supplementary Table 1 ). This is particularly significant for delivering sufficient power in practical applications. The achievement of comparably high specific capacitances for HGF in aqueous and organic electrolytes suggests that our HGF is distinct from traditional porous carbon materials such as activated carbon, activated graphene, templated carbon and carbide-derived carbon, which usually exhibit 20–40% lower specific capacitance in organic electrolyte than in aqueous electrolyte, with a relatively low specific capacitance in organic electrolytes (<180 F g −1 ) in spite of their high specific surface area (1,000–3,000 m 2 g −1 ) (refs 3 , 4 , 5 , 6 , 12 , 30 ). This is largely because these porous carbon materials usually have abundant wormlike tortuous pore channels, a large portion of which cannot be efficiently accessed by the large organic electrolyte ions [3] , [4] , [5] , [6] , and thus are less electrochemically active. In contrast, the HGFs here have several unique features to ensure a high capacitance both in aqueous and organic electrolytes: (1) The graphene building block has an ideal two-dimensional flat surface and an ultrahigh theoretical specific surface area of 2,630 m 2 g −1 . The 3D self-assembly of holey graphene sheets produces a unique porous network structure with the two-dimensional graphene surface readily accessible by electrolyte ions. (2) The HGFs are fully hydrated as prepared and can be readily infiltrated with organic electrolyte through a solvent exchange process to ensure the entire surface area is naturally wetted by electrolyte and accessible by the electrolyte ions. (3) The nanopores in the holey graphene sheet have sizes comparable to or larger than those of organic electrolyte ions and can function as the ion transport shortcuts between neighbouring layers of graphene to greatly speed up the ion transport process for improved rate performance. Previous studies on chemically reduced graphene indicate that ESR values achieved in organic versus aqueous electrolytes could differ substantially (up to 10–20 times) [10] . In contrast, our EIS studies demonstrate that the ESR values of HGF electrodes show a much smaller difference in organic versus aqueous electrolyte ( Supplementary Fig. 9 ), confirming that the HGF electrodes would be well suited for organic electrolyte. Furthermore, we have investigated the impact of different compression ratio (packing density) on the capacitive performance. Our studies demonstrates that a large compression ratio causes a much smaller degradation to the gravimetric capacitance and rate capability of HGF-ECs than it does to the non-holey GFs ( Supplementary Fig. 10 ), further highlighting that the unique hierarchical porosity in HGF is particularly important for retaining high specific capacitance and excellent rate performance under highly compressed conditions, which is essential for simultaneously achieving high gravimetric and volumetric capacitances. Together, our studies have demonstrated a new EC electrode design by creating a highly interconnected 3D HGF with superior electrical conductivity, exceptional mechanical flexibility and unique hierarchical porosity, which can ensure efficient electron and ion transport to enable the HGF-ECs with both the highest gravimetric and volumetric energy densities. Importantly, the overall energy density achievable in these HGF-ECs is comparable to traditional lead acid battery, and with much higher power density. The achievement of such high energy density in HGF-ECs bridges the gap between traditional capacitors and batteries, and can open up exciting opportunities for mobile power supply in a wide range of applications, including electrical vehicles and mobile electronics. Preparation of HGFs and GFs GO was prepared by oxidation of natural graphite powder according to the modified Hummers’ method [33] , [34] . HGFs were prepared based on the following procedure. A 1 ml diluted H 2 O 2 aqueous solution (0.3% H 2 O 2 ) was added into 10 ml 2 mg ml −1 GO aqueous dispersion in a 25 ml Teflon-lined autoclave. The mixture was sealed and heated at 180 °C for 6 h and naturally cooled down to room temperature and the as-prepared HGF was taken out with a pair of tweezers and immersed in 1 M sodium ascorbate aqueous solution at 100 °C for 2 h for further reduction. The HGF was lastly immersed in pure water to remove any impurities for the following experiments. GFs were prepared using the same procedure without adding any H 2 O 2 . The yield of HGFs compared with non-holey GFs is ~74%. In control experiments, 3 and 30% H 2 O 2 aqueous solution of the same volume (1 ml) were used to investigate the effect of H 2 O 2 concentration on the chemical etching of GO sheets. Fabrication of HGF- and GF-ECs Slices of HGF with a thickness of ~1 mm were first cut from the as-prepared cylindrical HGFs. For assembly of ECs with aqueous electrolyte: the HGF slices were immersed in 6.0 M KOH aqueous electrolyte for 12 h under stirring to exchange their interior water with electrolyte. For assembly of ECs with organic electrolyte: the HGF slices were first immersed in pure ionic liquid EMIMBF 4 under vacuum at 100 °C for 12 h to exchange their interior water with EMIMBF 4 and then transferred to a EMIMBF 4 /AN solution with a weight ratio of 1:1 for another 12 h. Subsequently, the HGF slices solvated with aqueous and organic electrolytes were placed on the platinum or aluminium foils, respectively, and compressed using hydraulic press at a rate of ~0.5 cm min −1 during which the squeezed electrolytes were removed by filter papers. The samples were kept under a 150-MPa pressure for 1 min to form ~14 μm well-adhered films on the metal foils. Next, two same HGF films (both with a net-weight of ~1 mg and an areal mass of ~1 mg cm −2 ) on separate metal foils were directly used as electrodes without any other additives or further treatments such as drying and thermal annealing, and separated by an ion-porous separator (Celgard 3501) soaked with electrolytes. All the components were assembled into a layered structure and tightly sealed by parafilm for electrochemical measurements. The GF-ECs were fabricated using the similar methods. The assembly of ECs with EMIMBF 4 /AN electrolyte was done in a glove box filled with Ar. Thicker film electrodes with an areal mass loading of 10 mg cm −2 in ECs were prepared by compressing thicker HGF slices with a thickness of ~1 cm under the same pressure. To determine the packing density, we calculated the volume by measuring the radius ( r ) and thickness ( h ) of the compressed HGF film ( V = h × π × r 2 ) and directly weighed the net mass of the vacuum dried HGF. We can thus obtain the packing density by dividing the net mass by the volume of the HGF film. Structural characterization and analysis The morphologies of HGFs were characterized by s.e.m. (JEOL 6700) and TEM (FEI CM120). X-ray diffraction were collected on a Panalytical X'Pert Pro X-ray Powder Diffractometer with Cu-Kα radiation. MB dye adsorption method was employed to measure the specific surface areas of HGFs and GFs. MB adsorption is a standard method for measuring the specific surface area of graphitic materials, with 1 mg of adsorbed MB molecules covering 2.54 m 2 of surface area [35] . The surface areas were calculated by adding a piece of HGF or GF into a standard concentration of MB in DI water for a total of 24 h to reach adsorption equilibrium. The MB concentration was determined by analysing the supernatant through UV–vis spectroscopy at a wavelength of 665 nm and compared with the initial standard concentration of MB before interacting with HGF or GF. Electrochemical characterization and analysis All the electrochemical experiments were carried out using VersaSTAT 4 from Princeton Applied Research. The EIS measurements were performed at open circuit potential with a sinusoidal signal over a frequency range from 100 kHz to 10 mHz at an amplitude of 10 mV. The cycle life tests were conducted by galvanostatic charge/discharge measurements. For the leakage current test, the HGF-ECs were first charged to 3.5 V at 10 mA and then the potential was kept at 3.5 V for 2 h while acquiring the current data. The gravimetric capacitances ( C wt ) of HGF and GF electrodes derived from galvanostatic discharge curves were calculated based on the following formula: C wt =2( I Δ t )/( m Δ V ), where I is the constant discharge current, Δ t is the time for a full discharge, m is the net mass of one electrode and Δ V represents voltage drop on discharging (excluding the V drop ). The corresponding volumetric capacitances ( C vol ) of HGF and GF electrodes were calculated using: C vol = C wt × ρ , where ρ is the packing density of graphene in HGF or GF films. The gravimetric ( E wt ) and volumetric ( E vol ) energy density against two electrodes in device were calculated using the following formula: E wt = C wt V 2 /8 and E vol = C vol V 2 /8, respectively, where V is the operating voltage (obtained from the discharge curve subtracted by the V drop ). The areal energy density of the device was calculated by: E area = E wt × 2 × M area , where M area is the areal mass loading of graphene in one electrode. The total energy density of the device was calculated by: E total = E wt × M total , where M total is the total mass of graphene in two electrodes. The gravimetric or volumetric energy density against the entire EC stack ( E stack ) was obtained based on the following formula: E w-stack = E wt × f w-electrode or E v-stack = E vol × f v-electrode , where f w-electrode is calculated by dividing the net mass of two electrodes by the total mass of the device stack or f v-electrode is calculated by dividing the thickness of the two electrodes by the total thickness of the device stack. The entire device stack includes two electrodes, two current collectors, electrolyte, one separator and/or parafilm packaging. The thickness and areal mass of one membrane separator with electrolyte are ~30 μm and ~3 mg cm −2 ; the thickness and areal mass of one aluminium current collector are 20 μm and 5.4 mg cm −2 ; the thickness and areal mass of total wrapped parafilm package are ~100 μm and ~10 mg cm −2 ; the thickness and areal mass of one thick electrode with electrolyte are ~140 μm and ~20 mg cm −2 . The gravimetric and volumetric stack energy densities were normalized by the total mass and volume of the entire device with only consideration of electrode area, which is similar to the approach used in recent reports [13] , [16] . The various power densities of the device ( P ) were calculated from the following formula: P = E /Δ t , where Δ t is the discharge time. R ESR is the ESR of the device, which was calculated via dividing the voltage drop ( V drop ) at the beginning of the discharge by the applied constant current ( I ) using the formula: R ESR = V drop /2 I . How to cite this article: Xu, Y. et al . Holey graphene frameworks for highly efficient capacitive energy storage. Nat. Commun. 5:4554 doi: 10.1038/ncomms5554 (2014).